Ionic polypeptides with unusual helical stability Water-soluble peptides that adopt stable helical conformations are attractive motifs because of their importance in basic science and their broad utility in medicine and biotechnology. Incorporating charged amino-acid residues to improve peptide solubility, however, usually leads to reduced helical stability because of increased side-chain charge repulsion, reduced side-chain hydrophobicity and the disruption of intramolecular hydrogen bonding. Here, we show that water-soluble, ultra-stable α-helical polypeptides can be produced by elongating charge-containing amino-acid side chains to position the charges distally from the polypeptide backbone. The strategy has been successfully applied to the design and synthesis of water-soluble polypeptides bearing long, charged side chains and various functional moieties that possess unusual helical stability against changing environmental conditions, including changes in the pH and temperature and the presence of denaturing reagents. The α-helix, the most prevalent type of secondary structure found in proteins, forms the cornerstone of the three-dimensional architecture of proteins and regulates numerous biological activities [1] . As a motif with a unique folding/unfolding property and a rigid rod-like morphology, the α-helix has been the subject of intense study and has been broadly used as a building block in the design of therapeutics and molecular assemblies [2] , [3] , [4] , [5] , [6] , [7] , [8] , [9] , [10] , [11] , [12] . Polypeptides bearing an α-helical conformation can be made entirely of hydrophobic amino acids with high helical propensities (for example, Ala and Leu) [13] , [14] , [15] . However, the usefulness of these structures is limited because of their poor aqueous solubility and processability. In the past, interest has been largely focused on the design and synthesis of water-soluble α-helical polypeptides or peptide motifs that usually contain a handful of charged amino acids (for example, Glu or Lys). Yet, the incorporation of charged residues into polypeptides often results in increased side-chain electrostatic repulsion [3] , [16] , [17] , [18] , which tends to destabilize the helical conformation. In the extreme context in which the polypeptides are made exclusively of amino acids bearing charged side chains, such as poly( L -glutamate) (PLG) or poly( L -lysine) (PLL), they adopt random coil conformations when their side chains are charged. As increasing the water solubility by introducing charge groups and enhancing the helical stability of polypeptides are often contradictory to each other, it has been a routine strategy to integrate both water-soluble and helix-stabilizing motifs in the peptide structure to design water-soluble helical peptides. Often, peptides are designed to have the charged amino-acid residues placed on one side of the helix surface and the residues responsible for stabilizing the helix through side-chain hydrophobic interactions [18] , salt bridges [19] or tethering [20] placed on the opposite side of the helix surface. These strategies require the design of peptides with specific sequences and/or involve tedious chemistries of polypeptide side chains that are typically difficult to control. For polypeptides made by polymerization rather than through stepwise synthesis, the above-mentioned helix-stabilization strategies cannot be applied. Water-soluble polypeptides that adopt stable α-helical conformations have long been sought after. Tremendous efforts have been focused on introducing neutrally charged, hydrophilic functional groups [21] or moieties [22] . For instance, poly( N -hydroxyalkyl- L -glutamine) [21] , derived from aminolysis of poly( L -glutamate esters), was found to be water soluble because of its pendant hydroxyl groups. It adopts a moderately high helical structure (up to ∼ 65% helicity) in aqueous solution [21] . Deming and co-workers reported the synthesis of PLL-containing pendant oligoethyleneglycol moieties using the ring-opening polymerization (ROP) of oligoethyleneglycol-containing lysine N -carboxyanhdyride (NCA) [22] . The resulting oligoethyleneglycol-graft PLL showed excellent water solubility and up to ∼ 100% helical structure in pH 7 water at 25 °C. These polypeptides were designed in a manner to introduce water-soluble motifs on an α-helical structure in the absence of electrostatic perturbations. To our knowledge, charged, water-soluble polypeptides that adopt stable α-helical conformations, that is, α-helical polypeptide electrolytes (αHPEs), have never been reported. When analysing helix-forming amino acids, it can be found that Ala and its three analogues, α-aminobutyric acid, norvaline and norleucine ( Fig. 1a ), have identical helical propensities [23] , indicating that the linear elongation of an amino-acid side chain with hydrocarbons does not affect its helix-forming capability. When a charged group (for example, COO − or NH 3 + ) is placed at the termini of the hydrocarbon side chains of these amino acids, however, substantially reduced amino-acid helix propensity scales are noted [24] . Interestingly, the helix propensity of Asp − , Glu − , Lys + and Arg + , the four charged natural amino acids with straight side chains ( Fig. 1b ), is strongly correlated with the length of the hydrocarbon side chain; the longer the hydrocarbon side chains (the further away the charge is from the backbone), the higher the helix-forming propensity. Their helical propensities are in the order of Arg + >Lys + >Glu − >Asp − , where the charge is 6, 5, 4 or 3 σ-bonds away from the peptide backbone, respectively ( Fig. 1b ) (ref. 24 ). We reasoned that the differences in their helix-forming propensities could be partly due to the differences in charge density on the helical surfaces, with the poly(Arg + ) helix being the lowest (the largest helical surface area, the weakest electrostatic repulsion) and poly(Asp − ) being the highest (the smallest helical surface area, the strongest electrostatic repulsion) if they are both formed ( Fig. 1c ). We postulated that when the charge is moved further away from the peptide backbone to reduce the overall charge density on the helical surface and charge repulsion, at some point the charge may have a negligible effect on the helical propensity of amino acids with long, straight side chains. As a result, these polypeptides with charges that are distally situated from the peptide backbone on a hydrophobic side chain may simultaneously maintain water solubility and stable helical structures ( Fig. 1d ). 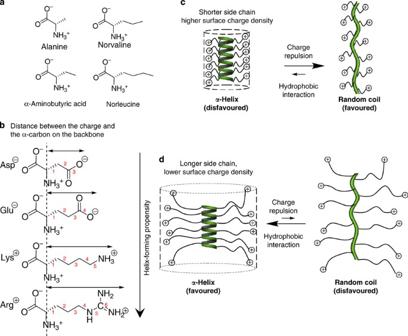Figure 1: Amino acids and their helix-forming properties. (a) Illustration of amino acids containing linear hydrocarbon side chains with variable lengths. (b) Illustration of four amino acids with charged side chains (Asp, Glu, Lys and Arg) and the correlation of their helix-forming propensity with the distance between the side-chain charge and the α-carbon. (c) Illustration of polypeptides with short, charged side chains and the postulated helix-to-random coil transition because of side-chain charge repulsion. (d) Illustration of polypeptides with long, charged side chains and postulated random coil-to-helix transition because of reduced side-chain charge repulsion. Figure 1: Amino acids and their helix-forming properties. ( a ) Illustration of amino acids containing linear hydrocarbon side chains with variable lengths. ( b ) Illustration of four amino acids with charged side chains (Asp, Glu, Lys and Arg) and the correlation of their helix-forming propensity with the distance between the side-chain charge and the α-carbon. ( c ) Illustration of polypeptides with short, charged side chains and the postulated helix-to-random coil transition because of side-chain charge repulsion. ( d ) Illustration of polypeptides with long, charged side chains and postulated random coil-to-helix transition because of reduced side-chain charge repulsion. Full size image In this study, we prepared a series of PLG analogues with extented, hydrophobic side chains bearing a terminal, positively charged amine group. When the amine group was placed 11 σ-bonds away from the polypeptide backbones, the corresponding polypeptide bearing positive charges on its side chains indeed showed remarkable α-helical conformations crossing a broad range of pH (from 1 to 10). This design principle has been applied to the synthesis of a handful of polypeptides with similar side-chain strucutres and has been confirmed as these polypeptides all possess α-helical conformations with unusual helical stability against changing environmental conditions. Poly( L -glutamates) with charged and long side chains To test this hypothesis, we prepared a 57mer of poly(γ-(3-aminopropyl)- L -glutamate) (PAPG 57 ), a 50mer of poly(γ-(5-aminopentanyl)- L -glutamate) (PAPTG 50 ) and a 57mer of poly(γ-(6-aminohexyl)- L -glutamate) (PAHG 57 ) through the ROPs of γ-benzyl- L -glutamate N -carboxyanhydride (Glu-NCA) [25] , [26] , [27] followed by removing the benzyl ester PBLG side chains and grafting the corresponding amino alcohol to the pendant carboxylate groups of PLG by the formation of ester bonds ( Fig. 2a , Supplemenary Figs S1–S3 ). PAPG 57 , PAPTG 50 and PAHG 57 contain hydrophobic side chains with different lengths and a terminal, charged amine group (−NH 3 + ) situated 8, 10 and 11 σ-bonds, respectively, away from its backbone. Compared with the circular dichroism (CD) spectrum of a 75mer of PLL (PLL 75 ) at pH 3, which is known to adopt a random coil conformation, the CD spectrum of PAPG 57 at pH 3 showed some characteristics of an α-helical conformation ( Fig. 3a ). A minimum at 222 nm with a molar ellipticity [ θ ] 222 ) value of −3,100 cm 2 deg dmol −1 was observed, which corresponds to ∼ 16% of helical content [28] ; the other expected minimum around 208 nm was not obvious. The characteristic double minima of the CD spectrum of an α-helical conformation became more obvious in PAPTG 50 with its helical content at pH 3 increased to ∼ 29% with a [ θ ] 222 value of −7,400 cm 2 deg dmol −1 . For PAHG 57 that has the largest space between the charged, terminal amine group and the polypeptide backbone, it adopts an α-helical conformation, as shown in its CD spectrum with characteristic double minima at 222 and 208 nm and has a helical content of 45%. Apparently, the hypothesis of creating water-soluble, charged, helical polypeptides by placing charges distally situated from the peptide backbone is demonstrated to be correct. 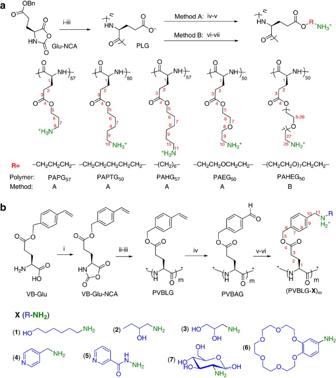Figure 2: Synthesis of polypeptides with charged side chains. (a) Synthesis of PAPG, PAPTG, PAHG, PAEG and PAHEG. The brief reaction condition of each step was listed below: (i) hexamethyldisilazane (HMDS)/DMF; (ii) CBZ-Cl; (iii) HBr; (iv) OH-R-NH(Boc), BOP-Cl; (v) HCl; (vi) OH-R-N3, BOP-Cl; (vii) 1. PPh3, CHCl3; 2. NH3-H2O. (b) Synthesis of PVBLG-X. The brief reaction condition of each step was listed below: (i) phosgene; (ii) HMDS/DMF/nitrobenzene; (iii) benzyl chloroformate/diisopropyl ethyl amine/tetrabutylammonium floride; (iv) O3/CHCl3/−78 °C; v.X/[H] (X=1–7); (vi) HCl. Figure 2: Synthesis of polypeptides with charged side chains. ( a ) Synthesis of PAPG, PAPTG, PAHG, PAEG and PAHEG. The brief reaction condition of each step was listed below: (i) hexamethyldisilazane (HMDS)/DMF; (ii) CBZ-Cl; (iii) HBr; (iv) OH-R-NH(Boc), BOP-Cl; (v) HCl; (vi) OH-R-N 3 , BOP-Cl; (vii) 1. PPh 3 , CHCl 3 ; 2. NH 3 -H 2 O. ( b ) Synthesis of PVBLG- X . The brief reaction condition of each step was listed below: (i) phosgene; (ii) HMDS/DMF/nitrobenzene; (iii) benzyl chloroformate/diisopropyl ethyl amine/tetrabutylammonium floride; (iv) O 3 /CHCl 3 /−78 °C; v. X /[H] ( X = 1 – 7 ); (vi) HCl. 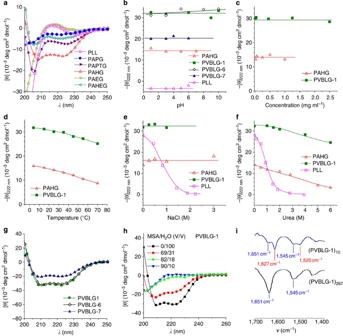Figure 3: Characterization of charged polypeptides. PAHG and PVBLG-X, polypeptides with long, charged, hydrophobic side chains, adopt very stable α-helica conformations at low pH, at elevated temperature, or in solution containing high concentration of salt or denaturing agents (for example, urea or MSA). (a) CD spectra of various polypeptides bearing charged side chains (PAPG, PAPTG, PAHG, PAEG and PAHEG) in aqueous solution at pH 3. The mean residue molar ellipticity was calculated by following literature-reported formulas: Ellipticity ([θ]222 nmin cm2deg dmol−1)=(millidegrees×mean residue weight)/(path length in millimetres×concentration of polypeptide in mg ml−1)39,40. (b) The pH dependence of the residue molar ellipticity at 222 nm for (PAHG)57, (PVBLG-1)60, (PVBLG-6)44, (PVBLG-7)40and (PLL)75. (c) Concentration dependence of residue molar ellipticity at 222 nm for (PAHG)57and (PVBLG-1)60at pH 3. (d) Temperature dependence of residue molar ellipticity at 222 nm for (PAHG)57and (PVBLG-1)60at pH 3. (e) Salt concentration dependence of residue ellipticity at 222 nm for (PAHG)57and (PVBLG-1)60at pH 3 and (PLL)75at pH 10. (f) The helical stabilities of (PAHG)57and (PVBLG-1)60at pH 3 and (PLL)75at pH 10 in the presence of urea. (g) CD spectra of (PVBLG-1)60, (PVBLG-6)44and (PVBLG-7)40. (h) CD spectra of (PVBLG-1)60in a mixed solvent of MSA and H2O. (i) Fourier-transform infrared spectra of (PVBLG-1)10and (PVBLG-1)267. Infrared spectra were recorded on a Perkin Elmer 100 serial FTIR spectrophotometer (Perkin Elmer) equipped with universal attenuated total reflectance (ATR), which enabled the analysis of PVBLG in powder form. (PVBLG-1)10and (PVBLG-1)267were purified by dialysis and lyophilized. The fluffy samples were placed on the crystal of the sampling accessory for ATR analysis. Full size image Figure 3: Characterization of charged polypeptides. PAHG and PVBLG- X , polypeptides with long, charged, hydrophobic side chains, adopt very stable α-helica conformations at low pH, at elevated temperature, or in solution containing high concentration of salt or denaturing agents (for example, urea or MSA). ( a ) CD spectra of various polypeptides bearing charged side chains (PAPG, PAPTG, PAHG, PAEG and PAHEG) in aqueous solution at pH 3. The mean residue molar ellipticity was calculated by following literature-reported formulas: Ellipticity ([ θ ] 222 nm in cm 2 deg dmol −1 )=(millidegrees×mean residue weight)/(path length in millimetres×concentration of polypeptide in mg ml −1 ) [39] , [40] . ( b ) The pH dependence of the residue molar ellipticity at 222 nm for (PAHG) 57 , (PVBLG- 1 ) 60 , (PVBLG- 6 ) 44 , (PVBLG- 7 ) 40 and (PLL) 75 . ( c ) Concentration dependence of residue molar ellipticity at 222 nm for (PAHG) 57 and (PVBLG- 1 ) 60 at pH 3. ( d ) Temperature dependence of residue molar ellipticity at 222 nm for (PAHG) 57 and (PVBLG-1) 60 at pH 3. ( e ) Salt concentration dependence of residue ellipticity at 222 nm for (PAHG) 57 and (PVBLG- 1 ) 60 at pH 3 and (PLL) 75 at pH 10. ( f ) The helical stabilities of (PAHG) 57 and (PVBLG- 1 ) 60 at pH 3 and (PLL) 75 at pH 10 in the presence of urea. ( g ) CD spectra of (PVBLG- 1 ) 60 , (PVBLG- 6 ) 44 and (PVBLG- 7 ) 40 . ( h ) CD spectra of (PVBLG- 1 ) 60 in a mixed solvent of MSA and H 2 O. ( i ) Fourier-transform infrared spectra of (PVBLG- 1 ) 10 and (PVBLG- 1 ) 267 . Infrared spectra were recorded on a Perkin Elmer 100 serial FTIR spectrophotometer (Perkin Elmer) equipped with universal attenuated total reflectance (ATR), which enabled the analysis of PVBLG in powder form. (PVBLG- 1 ) 10 and (PVBLG- 1 ) 267 were purified by dialysis and lyophilized. The fluffy samples were placed on the crystal of the sampling accessory for ATR analysis. Full size image PAHG 57 showed remarkable pH-independent helical stability at pH values ranging from 1 to 10, with −[ θ ] 222 value at 14,000 cm 2 deg dmol −1 for pH 1 and at 14,200 cm 2 deg dmol −1 for pH 10 (≈44–45% helical content; Fig. 3b , Supplementary Fig. S4 ). Further increases in pH (pH >11) resulted in deprotonation of the positively charged amino group on the side chain and a decreased solubility of PAHG 57 . PAHG 57 also showed a lack of concentration dependence of its –[ θ ] 222 and –[ θ ] 208 values in helix-forming conditions, suggesting that it remains monomeric in solution ( Fig. 3c , Supplementary Fig. S5 ). PAHG 57 showed temperature-dependent helical stability as its –[ θ ] 222 value decreased 45% from 15,900 cm 2 deg dmol −1 at 4 °C to 8,700 cm 2 deg dmol −1 at 70 °C ( Fig. 3d , Supplementary Fig. S6 ). It exhibited remarkable stability against the change in the NaCl concentration and remained nearly unchanged in its −[ θ ] 222 value when the NaCl concentration was increased from 0 to 4.7 M at pH 3 at 25 °C, a concentration for which all of the charges should have been screened, which is distinctly different from PLL 75 ( Fig. 3e , Supplementary Fig. S7 ). These experiments further demonstrate that the surface charges of PAHG 50 have minimal effects on its helical stability. The helical conformation of PAHG 57 was gradually disrupted at increased concentrations of strong denaturing reagents such as urea and methanesulfonic acid (MSA) ( Fig. 3f , Supplementary Figs S8–S9 ). To elucidate the effect of the side-chain hydrophobicity and the charge on the formation and stabilization of α-helical conformations, we synthesized a 50mer of poly(γ-(2-aminoethyl)-ethyleneglycol- L -glutamate) (PAEG 50 ) ( Fig. 2a , Supplementary Fig. S10 ). PAEG 50 has exactly the same structure as PAPTG 50 except that one 'CH 2 ' unit of PAPTG 50 was replaced by an 'O' in PAEG 50 , which makes PAEG more hydrophilic than PAPTG. The CD analysis showed that PAEG 50 adopts a random coil structure at pH 3 when the terminal amine is protonated ( Fig. 3a ), which underscores the importance of the hydrophobicity of the side chains connecting the terminal charge and the backbone on the stabilization of the α-helical conformation. Interestingly, when the side chain of PAEG 50 was elongated by inserting a hydrophilic, hepta(ethylene glycol) to further extend the charged amine group, a random coil-to-helix transition was observed and the resulting poly((γ-(2-aminoethyl)-heptaethyleneglycol)- L -glutamate) (PAHEG 50 ) ( Supplementary Fig. S11 ) adopts an α-helical conformation at pH 3. These experiments suggest that the reducing helical surface charge density (reducing side-chain charge repulsion) is crucial to the stabilization of α-helical conformation. Design, synthesis and conformation analysis of poly(γ-(4-vinylbenzyl)- L -glutamate)s Motivated by this discovery, we next tested whether this helix-stabilization strategy could be generally applied to designing water-soluble, αHPEs that contain charged secondary amines with various functional moieties attached to the amine. To avoid the harsh deprotection chemistry and low conjugation activity illustrated in Figure 2a , we attempted and successfully developed a highly efficient conjugation strategy that involves the ROP of γ-(4-vinylbenzyl)- L -glutamate NCA (VB-Glu-NCA) to yield poly(γ-(4-vinylbenzyl)- L -glutamate) (PVBLG, Supplementary Fig. S12 ) followed by the formation of poly(γ-(4-aldehydebenzyl)- L -glutamate) (PABLG, Supplementary Fig. S13 ) through the ozonolysis of PVBLG, and hydroamination of the PABLG with 6-amino-1-hexanol ( 1 ) to give the desired products (PVBLG- 1 ) m , where ' m ' corresponds to the degree of VB-Glu-NCA polymerization ( Fig. 2b , Supplementary Fig. S14 ). The positive charge of (PVBLG- 1 ) m was placed exactly 11 σ-bonds away from its backbone, just like PAHG. VB-Glu-NCA can be readily prepared and purified by crystallization on a multi-gram scale [29] , [30] and can be polymerized in a highly controlled manner to yield PVBLGs using N -trimethylsilyl ( N -TMS) amine initiators previously developed by our group ( Fig. 4a ) (ref. 25 ). The obtained M n values of the PVBLGs were in excellent agreement with the expected molecular weights (MWs; <5–15% MW deviation), and the polydispersities (PDIs) of the PVBLGs were all below 1.10 ( Fig. 4a ). Such hexamethyldisilazane-mediated VB-Glu-NCA polymerizations are highly reproducible. We repeated the polymerization at a monomer-to-initiatior (VB-Glu-NCA/hexamethyldisilazane) ratio of 100:1 in three separate experiments using the VB-Glu-NCA from different batches, the obtained average M n value was 24.3±2.7×10 3 g mol −1 , which was in almost perfect agreement with the expected MW (24.5×10 3 g mol −1 ). The MWs of PVBLG showed linear correlation with the conversions of VB-Glu-NCA and agreed perfectly with the expected MWs ( Fig. 4b ), demonstrating that PVBLG chains were propagated through living chain ends [27] . PVBLGs are very soluble in common organic solvents (for example, THF, CHCl 3 and DMF), which facilitates their side-chain modification to yield (PVBLG- 1 ) m with over 95% grafting efficiency (entries 1–6 in Table 1 ). 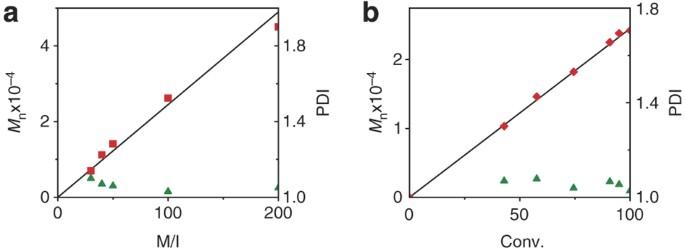Figure 4: Controlled polymerization of VB-Glu-NCA. (a) The molecular weights (MWs) and polydispersities (PDIs) of PVBLGs derived from the ROP of VB-Glu-NCA initiated by hexamethyldisilazane at various monomer-to-initiatior (M/I) ratios in DMF (containing 5% nitrobenzene). (b) The MWs and PDIs at various VB-Glu-NCA conversions at an M/I ratio of 100:1 in DMF (containing 5% nitrobenzene). The black curve indicates the correlation of the theoretical MW with the M/I ratio inaor with the conversion of VB-Glu-NCA inb; the obtained MWs are denoted as the red squares in bothaandb; the PDIs are denoted as the green triangules in bothaandb. Figure 4: Controlled polymerization of VB-Glu-NCA. ( a ) The molecular weights (MWs) and polydispersities (PDIs) of PVBLGs derived from the ROP of VB-Glu-NCA initiated by hexamethyldisilazane at various monomer-to-initiatior (M/I) ratios in DMF (containing 5% nitrobenzene). ( b ) The MWs and PDIs at various VB-Glu-NCA conversions at an M/I ratio of 100:1 in DMF (containing 5% nitrobenzene). The black curve indicates the correlation of the theoretical MW with the M/I ratio in a or with the conversion of VB-Glu-NCA in b ; the obtained MWs are denoted as the red squares in both a and b ; the PDIs are denoted as the green triangules in both a and b . Full size image Table 1 Synthesis and conformation analysis of PVBLG- X . Full size table (PVBLG- 1 ) 60 is highly water soluble at pH 1–10 (>40 mg ml −1 ) and adopts an α-helical conformation with a –[ θ ] 222 value of 32,600 cm 2 deg dmol −1 for pH values as low as 1 ( Fig. 3g , Supplementary Fig. S15 ). The high helical content of (PVBLG- 1 ) 60 as compared with PAHG 57 is presumably because of its increased side-chain hydrophobic interactions. The –[ θ ] 222 value of (PVBLG- 1 ) 60 remained unchanged when the solution's pH was increased from 1 to 10 ( Fig. 3b ). At further increased pH values, (PVBLG- 1 ) 60 became less soluble because of deprotonation of its charged secondary amine groups. As with PAHG 57 , (PVBLG- 1 ) 60 showed a lack of concentration dependence of its –[ θ ] 222 and –[ θ ] 208 values in helix-forming conditions, suggesting that it remains monomeric in solution ( Fig. 3c , Supplementary Fig. S16 ). It has excellent helical stability against elevated temperatures, with its –[ θ ] 222 value decreasing 21% from 31,700 cm 2 deg dmol −1 at 4 °C to 25,100 cm 2 deg dmol −1 at 70°C ( Fig. 3d , Supplementary Fig. S17 ), and against helix-destabilizing conditions such as high concentrations of NaCl ( Fig. 3e ), urea ( Fig. 3f ) and methanesulfonic acid (MSA; Fig. 3h; Supplementary Figs S18–S20 ). PVBLG- 1 has unprecedented helical stability against any known α-peptides and can maintain 76 and 58% of its original helical contents in 6 M urea and 69% MSA, respectively. Interestingly, the urea-mediated helix-destabilization experiments do not show the typical helix-to-random coil two-state transition, whereas the MSA-induced denaturation experiments do seem to be consistent with the two-state model with an isodichroic point around 203 nm (ref. 31 ; Supplementary Figs S19–S20 ), suggesting the denaturization mechanisms in urea and MSA are different. The –[ θ ] 222 value of low-MW PVBLG- 1 's (below 60mer) is strongly correlated with the length of the polymer, and is gradually plateaued at around 32,000 ∼ 33,000 cm 2 deg dmol −1 (>90% helical contents) for PVBLG- 1 's with MWs beyond 60mer ( Table 1 ; Supplementary Fig. S21 ). PVBLG- 1 's with very low MW, such as (PVBLG- 1 ) 10 , have mixed conformations containing both α-helices and β-sheets in solid state based on the Fourier-transform infrared analysis ( Fig. 3i ). We exploited this strategy for the synthesis of PVBLG αHPEs with various other motifs on the helix surface ( Supplementary Figs S22–S27 ). Amine-containing alcohols (1-amino-2-butanol ( 2 ) and 3-amino-1,2-dipropanol ( 3 )), pyridines (4-(aminomethyl)pyridine ( 4 ) and nicotinic hydrazide ( 5 )), a crown ether (4-aminobenzo-18-crown-6 ( 6 )) and a carbohydrate ( D -glucosamine ( 7 )) were selected to make the corresponding PVBLG- X ( X = 2 – 7 ) αHPEs. The grafting efficiencies for all of the PVBLG- X s are excellent (>95%), except for (PVBLG- 7 ) 40 , which has a grafting efficiency of 70% presumably because of the increased steric bulk of the carbohydrate molecules ( Table 1 ). All of the PVBLG- X s are water soluble and adopt α-helical conformations with minima at 208 and 222 nm for their CD spectra ( Fig. 3g and Supplementary Figs S28–S33 ). Interestingly, (PVBLG- 4 ) 40 and (PVBLG- 6 ) 44 showed comparable or even larger –[ θ ] 222 values and helical contents as compared with (PVBLG- 1 ) 40 , confirming our hypothesis that the physicochemical properties and size of the moieties attached to the amine situated distally from the polypeptide backbone have negligible effects on the helical stability of the αHPEs. PVBLG αHPEs containing pyridine, crown ether or sugar on the side chain all adopt very stable helical structures in water, demonstrating the robustness of this strategy in generating water-soluble rod-like αHPEs. It should be noted that the pyridine residues on the side chains of PVBLG- 4 are likely protonated at low pH (lower than the pKa of pyridine, which is around 5–6). Therefore, the CD spectrum of PVBLG- 4 recorded at pH 3, which showed characteristic two minima, suggests that polypeptides containing two charges per residue can still adopt stable helical conformation in aqueous solution ( Supplementary Fig. S31 ). PVBLG- 2 to - 7 also showed a helical stability similar to that of PVBLG- 1 against changes in the pH, temperature and salt and in the presence of denaturing reagents, as exemplified by (PVBLG- 6 ) 44 , which showed remarkable stability at various pH conditions ( Fig. 3b ). Polypeptide bearing charged side chains, such as PLG and PLL, typically adopt random coil conformations. These polypeptide electrolytes have been intensively studied for their chemicophysical properties and broadly used in various applications. For instance, they have been used as vehicles in drug and gene delivery [32] , [33] , as the building blocks of self-assembly [34] , as the water-soluble domains for preparing hydrogels for tissue engineering applications [12] and as the coating materials for surface modification [35] . In these applications, the polypeptides were simply treated as polymeric electrolytes; the capability of polypeptides to form rigid, rod-like α-helical structures, which differentiates polypeptides from many other polyelectrolytes, cannot be used because of the strong helix-destabilizing, side-chain electrostatic repulsions. We hypothesized that polypeptides bearing side-chain charges distally situated from the polypeptide backbones may simultaneously maintain water solubility (because of the charges) and stable helical structures (because of the reduced side-chain electrostatic repulsions ( Fig. 1d ). To demonstrate this hypothesis, we prepared PAPG 57 , PAPTG 50 and PAHG 57 , and compared their conformations against PLL, which is known to adopt random coil conformation in aqueous solution. The conformation analysis using CD clearly showed that elongating the polypeptide side chains to extend the charge away from polypeptide backbone can indeed allow helical conformation well maintained in polypeptide electrolytes. PAHG 57 that has the longest side chains separating the charge and polypeptide backbone adopts the highest helical content among these three tested polypeptides. We found that the hydrophobicity of the charged side chains also has significant effect on the helix stability. PAPTG 50 contains ∼ 29% of helical content, whereas PAEG 50 , which has exactly the same structure as PAPTG 50 except that one 'CH 2 ' unit of PAPTG 50 is replaced by an 'O' in PAEG 50 , and thus makes PAEG more hydrophilic than PAPTG, adopts completely random coil conformation ( Fig. 3a ). When polypeptide bearing hydrophilic, charged side chains, the space between the charge and backbone has to be sufficiently long to reduce the helix-destabilizing, electrostatic repulsion force in order for such polypeptide electrolytes to maintain some helical conformations, as shown in the case of PAHEG. However, without hydrophobic side chains to provide critical helix-stabilizing force, simply reducing side-chain electrostatic repulsion force can only give rise to polypeptide electrolytes with low helical contents, evidenced by the weak CD signal of PAHEG at 222 nm ( Fig. 3a ). To avoid the complex chemistry involved in the synthesis of poly( L -glutamate) analogues with long, charge-containing side chains as shown in Figure 2a , we attempted and successfully synthesized PVBLG- X , a class of new αHPEs that contain prolonged, hydrophobic side chains bearing charged amine moieties, using ROP of VB-Glu-NCA followed by the conversion of the pendant vinyl groups to aldehyde groups and subsequent reductive amination of aldehyde groups with the corresponding amino substrates (R-NH 2 ; Fig. 2b ). All PVBLG- X s we prepared adopt helical conformations because they contain a sufficiently long, hydrophobic spacer separating the positive charge and the polypeptide backbone. Interestingly, the size and the hydrophobicity/hydrophilicity of 'R' group do not seem to dramatically affect the stability of the helical conformation of PVBLG- X ( Table 1 ); our studies showed that 'R' can be hydrocarbon, alcohol, pyridine, saccharide or crown ether, and the corresponding PVBLG- X 's with charged side chains all adopt stable helical conformations in aqueous solution. These findings suggest that the critical helix-stabilizing force is controlled by the hydrophobic interaction of the side-chain segments immediately connected to the α-carbon of polypeptide, with length around 11 σ-bonds for both PAHG and PVBLG systems based on our experimental results. The charge-containing segments that are extended from the long, hydrophobic segments and distally situated from the polypeptide backbone show negligible effect on helical stability and are responsible for the water solubility of the polypeptides. Given that numerous primary amines are commercially available and can be used for the coupling with PABLG ( Fig. 2b ) to make PVBLG- X , a large library of PVBLG- X 's bearing various charged side chains can potentially be generated using this approach. In conclusion, we discovered that the length of the charged polypeptide side chains is crucial to the stability of the α-helical structures of polypeptide. When the side chains become sufficiently long and the charge groups are placed distally from the polypeptide backbone, the substantially reduced charge density on the helix surface causes the charge repulsion force to no longer be dominating and helix-disrupting. Our study indicated that polypeptides containing both hydrophobic and hydrophilic side chains with distally situated terminal charge groups can adopt helical conformations, but only polypeptides with long hydrophobic side chains show high helical contents. For polypeptide electrolytes with sufficiently long hydrophobic side chains (substantially reduced side-chain charge repulsion forces), side-chain hydrophobic interactions dominate to drive the formation of water-soluble, helical structures with remarkable helical stability despite changes in the pH or temperature and against various strong denaturing reagents. Our discovery may also explain why nature has not evolved to use amino acids with long, charged side chains as the building blocks for constructing proteins. As the reversibility of α-helix folding/unfolding is critical to many important biological processes, the incorporation of amino-acid residues bearing long, charged, hydrophobic side chains would have made the α-helix structure too stable to unfold. The simple polymerization method we have developed for producing helical, water-soluble polypeptides (PVBLG- X ) bearing various moieties should find various biological and biomedical applications. We also believe that the strategy of reducing helical surface charge density by incorporating amino acids with elongated, charged side chains can be generally applied to the design of sequence-specific peptides with highly stable helical conformations. Synthesis of PAHG. Synthesis of poly( L -glutamic acid) PLG 57 . Poly(γ-benzyl- L -glutamate) (PBLG) with a degree of polymerization of 57 (PBLG 57 ) was synthesized by following the procedure previously reported [27] . The M n is 12,500 g mol −1 and PDI ( M w / M n ) is 1.15 as characterized by gel permeation chromatograph (GPC). The deprotection of PBLG 57 was performed at 0 °C to give PLG 57 in quantitative yield by following a slightly modified, standard procedure [36] , [37] , [38] . The resulting polymer (500 mg) was treated with 2 M NaOH (10 ml) and then with CBZ-Cl (0.1 ml) for 16 h to protect the amino terminus of PLG with CBZ. The resulting PLG was acidified by 3 M HCl. The precipitates were purified subsequently by dialysis against deionized water followed by lyophilization. 1 H nuclear magnetic resonance (NMR; trifluoroacetic acid (TFA)- d , 500 MHz): δ 4.86 (1H, αH), 2.68 (2H, γH), 2.34 (1H, βH) and 2.19 (1H, βH). Synthesis of 6-( N -Boc-amino)-1-hexanol. 6-Amino-1-hexanol (1.17 g, 10 mmol) was dissolved in chloroform (15 ml) and stirred in an ice bath. (Boc) 2 O (2.25 g, 10.8 mmol) was added to the mixture in a small portion for about 5 min. The reaction mixture was stirred in the ice bath for another 2 h before the solvent was removed under vacuum. The crude product was recrystallized with hexane to give pure 6-( N -Boc amino)-1-hexanol (1.95 g, 90% yield). 1 H NMR (CDCl 3 , 500 MHz): δ 4.58 (s, 1H, N H ), 3.62 (t, 2H, J =8.0 Hz, −CH 2 CH 2 CH 2 C H 2 OH), 3.15 (t, 2H, J =7.5 Hz, BocNH CH 2 CH 2 ), 1.77 (S, 1H, –CH 2 CH 2 CH 2 CH 2 OH ), 1.60–1.30 (m, 17H, ( CH 3 ) 3 C(CO)NHCH 2 CH 2 CH 2 CH 2 CH 2 CH 2 OH). 13 C NMR (CDCl 3 , 500 MHz): δ 156.0, 79.0, 62.6, 40.3, 32.5, 30.2, 28.4, 26.3, 25.2. Synthesis of PAHG: PLG 57 (25 mg, 0.20 mmol Glu repeating unit), bis(2-oxo-3-oxazolidinyl)phosphonic chloride (BOP-Cl) (350 mg, 1.37 mmol), 4-dimethylaminopyridine (DMAP) (17 mg, 0.14 mmol), anhydrous triethylamine (0.2 ml, 1.4 mmol) and 6-( N -Boc amino)-1-hexanol (440 mg, 2 mmol) were added in anhydrous N -methylpyrrolidone (4 ml) under nitrogen in an ice bath. The conjugation reaction was allowed to proceed at 40–50 °C for 3 days. Ethyl acetate (30 ml) and a brine solution (20 ml) were added to the reaction mixture. The organic phase was washed with NaHCO 3 (1 M, 10 ml) and DI water (2×15 ml), dried with Na 2 SO 4 , and concentrated under vacuum. An oily residue was yielded, which was washed by ether (3×10 ml) to remove the excess 6-( N -Boc)-1-hexanol. The residue was dissolved in chloroform; TFA was added to the solution at room temperature. The mixture was stirred overnight, concentrated under vacuum to yield the deprotected crude product PAHG 57 . PAHG 57 was then dissolved in 3 M HCl, dialysed in DI water and lyophilized (22 mg, 43% overall yield). The grafting efficiency was 95% as calculated from 1 H NMR spectrum ( Supplementary Fig. S3 ). PAPG, PAPTG, PAEG and PAHEG were similarly prepared and characterized (see Supplementary Figs S1, S2, S10 and S11 , respectively). Synthesis of PVBLG- X ( X =1–7) . Synthesis of γ-(4-vinylbenzyl)- L -glutamate NCA (VB-Glu-NCA) γ-(4-Vinylbenzyl)- L -glutamate (VB-Glu) was synthesized by following a modified procedure [30] . VB-Glu (2.45 g, 10 mmol) was dried under vacuum for 2 h. This solid was suspended in anhydrous THF (30 ml). Phosgene (20% in toluene, 7 ml) was added under nitrogen to the solution dropwise for 5 min. The suspension was stirred at 50 °C for 2–3 h. The solvent was then removed under vacuum. The residue was dissolved in anhydrous THF in a glove box and centrifuged to remove the unreacted amino acid. The supernatant was combined and then the solvent was removed under vacuum. The residue was dissolved in THF (10 ml) followed by the addition of anhydrous ether (100 ml). The solution was cooled at −30 °C in the glove box. A dark oily residue was removed. The clear solution containing NCA was combined and concentrated. VB-Glu-NCA in white crystalline form (3.4 mmol, 1.0 g, 34%) was obtained through recrystallization three times using THF/hexane. 1 H NMR (CDCl 3 , 500 MHz): δ 7.40 (d, 2H, J =8.0 Hz, Ar H ), 7.30 (d, 2H, J =8 Hz, Ar H ), 6.73–6.67 (m, 2H, N H and C 6 H 4 C H =CH 2 ), 5.76 (d, 1H, J =17.5 Hz, C 6 H 4 CH=C H 2 ), 5.27 (d, 1H, J =11 Hz, C 6 H 4 CH=C H 2 ), 5.11 (s, 2H, Ar CH 2 ), 4.38 (t, 1H, J =6.0 Hz, C H CH 2 CH 2 COOCH 2 ), 2.58 (t, 2H, CH 2 CH 2 COOCH 2 ), 2.26 (m, 1H, CH 2 CH 2 COOCH 2 ), 2.12 (m, 1H, CH 2 CH 2 COOCH 2 ). 13 C NMR (CDCl 3 , 500 MHz): δ 172.4, 169.3, 151.9, 137.8, 136.1, 134.6, 128.6, 126.4, 114.6, 66.8, 56.9, 29.8, 26.8. Electrospray ionization mass spectrometry (ESI MS) analysis (with NaCl) calcd: m / z 289.2 (M); found: m / z 312.3 (M+Na). Analysis calculated for C 15 H 15 NO 5 : 62.29% C, 5.21% H, 4.84% N; found: 62.06% C, 5.12% H, 4.83% N. General procedure for the polymerization of VB-Glu-NCA. In a glove box, VB-Glu-NCA (29 mg, 0.1 mmol) was dissolved in the mixture of DMF (1 ml) and nitrobenzene (50 μl; nitrobenzene was used to inhibit potential radical reactions on vinyl group). The VB-Glu-NCA solution was added to a DMF solution of hexamethyldisilazane (20 μl, 0.1 mmol ml −1 ). The reaction mixture was stirred for 15 h at room temperature. An aliquot of the polymerization solution was diluted to 10 mg PVBLG per ml using DMF (containing 0.1 M LiBr), and then analysed by GPC. The M n and PDI were assessed by GPC ( M n =26,200 g mol −1 ; PDI ( M w / M n )=1.03). The remaining PVBLG was precipitated with ether (15 ml). The obtained PVBLG was sonicated for 5 min in ether and centrifuged to remove the solvent. After the sonication–centrifugation procedure was repeated two more times, PVBLG was collected and dried under vacuum (>95% yield). 1 H NMR (TFA- d , 500 MHz): δ 7.53 (d, 2H, J =7.0 Hz, Ar H ), 7.39 (d, 2H, J =7.0 Hz, Ar H ), 6.84 (dd, 1H, J 1 =11.0 Hz, J 2 18.0 Hz C 6 H 4 C H =CH 2 ), 5.91 (d, 1H, J =18.0 Hz, C 6 H 4 CH=C H 2 ), 5.43 (d, 1H, J =11.0 Hz, C 6 H 4 CH=C H 2 ), 5.26 (m, 2H, Ar CH 2 ), 4.80 (m, 1H, C H CH 2 CH 2 COOCH 2 ), 2.68 (m, 2H, CHCH 2 CH 2 COO), 2.30 (m, 1H, CH CH 2 CH 2 COO), 2.12 (m, 1H, CH CH 2 CH 2 COO) ( Supplementary Fig. S12 ). Synthesis of PABLG. PVBLG (10 mg) was dissolved in chloroform (10 ml) at −78 °C and O 2 was bubbled into the solution for 1 min, followed by bubbling of O 3 until the solution became blue. O 3 was then replaced by O 2 , which was bubbled into the solution for another 2 min until the solution became colourless. The solution was then degassed and back filled with nitrogen. Ph 3 P (26 mg) was then added to the mixture. The solution was stirred at room temperature for 2–3 h. The solvent was then removed under vacuum. The resulting PABLG was purified by sonicating the polymer in methanol (3×15 ml) to remove the unreacted Ph 3 P and other impurities. 1 H NMR (TFA- d , 500 MHz): δ 10.31 (1H, C H OC 6 H 4 ), 8.40 (d, 2H, J =7.0 Hz, ArH), 7.96 (d, 2H, J =7.0 Hz, ArH), 5.71 (2H, CHOC 6 H 4 CH 2 ), 5.21 (1H, CH CH 2 CH 2 CO 2 CH 2 ), 3.12 (2H, CHCH 2 CH 2 ), 2.75 (1H, CH CH 2 CH 2 ), 2.56 (1H, CH CH 2 CH 2 ) ( Supplementary Fig. S13 ). Synthesis of PVBLG- X ( X = 1 – 7 ). The PABLG (20 mg), amine (3–5 molar equiv. relative to the Glu repeating unit) and the reducing reagent (5–10 molar equiv. ; Table 1 ) were mixed in THF (3 ml; except for 7 with DMF was used as the solvent). The reaction mixtures were stirred at 50–60 °C for 24–72 h ( Table 1 ). The mixture was then poured into 3 M HCl (3 ml), followed by dialysis against water and lyophilization. The yields of the products PVBLG- X ( X = 1 – 7 ) were around 50–75% after dialysis. The grafting efficiencies were analysed by 1 H NMR ( Supplementary Figs S14, S22–S27 ). General procedure for the analysis of polypeptide conformations by CD. The CD experiments were conducted on a JASCO J-700 or a JASCO J-720 CD spectrometer. The polypeptide samples were generally prepared at concentrations of 0.01–0.1 mg ml −1 at pH 3 unless otherwise specified. The solution was placed in a quartz cell with a path length of 0.2 cm. The mean residue molar ellipticity of each polymer was calculated on the basis of the measured apparent ellipticity by following the literature-reported formulas: Ellipticity ([ θ ] in cm 2 deg dmol −1 )=(millidegrees×mean residue weight)/(path length in millimetres×concentration of polypeptide in mg ml −1 ) [39] , [40] . For the temperature-dependent experiments, the temperature of the sample chamber (where the quartz cell was placed) was controlled by a water bath (from 4 °C to 70 °C). The samples were equilibrated at the corresponding temperature for at least 10 min before the CD measurements. By following similar preparation method, the polymers were dissolved in DI water or in a solution containing NaCl, urea or MSA. For the pH-dependent experiments, the pH of the polymer solution was tuned by the addition of a concentrated HCl or NaOH solution. The α-helix contents of the polypeptides were calculated by the following equation: percentage of α-helix=(−[θ 222 ]+3,000)/39,000 [28] . How to cite this article: Lu, H. et al . Ionic polypeptides with unusual helical stability. Nat. Commun. 2:206 doi: 10.1038/ncomms1209 (2011).